Tyrosine sulfation in a Gram-negative bacterium Tyrosine sulfation, a well-characterized post-translation modification in eukaryotes, has not previously been reported in prokaryotes. Here, we demonstrate that the RaxST protein from the Gram-negative bacterium, Xanthomonas oryzae pv. oryzae, is a tyrosine sulfotransferase. We used a newly developed sulfotransferase assay and ultraviolet photodissociation mass spectrometry to demonstrate that RaxST catalyses sulfation of tyrosine 22 of the Xoo Ax21 (activator of XA21-mediated immunity) protein. These results demonstrate a previously undescribed post-translational modification in a prokaryotic species with implications for studies of host immune responses and bacterial cell–cell communication systems. Tyrosine sulfation is a common post-translational modification in eukaryotes [1] . In contrast to phosphorylation, which regulates processes that occur inside the cell [2] , sulfated proteins/peptides are typically directed outside the cell, where they modulate ligand–receptor interactions [3] . A notable example is the binding of the glycoprotein 120 (gp120) subunit of the human immunodeficiency virus (HIV), to the human chemokine co-receptors CD4 and CCR5 (ref. 4 ). Sulfation of tyrosine residues in the N-terminal segment of CCR5 seems to be critical for both HIV-1 entry and binding of gp120-CD4 complexes [5] . In plants, the sulfated peptide, phytosulfokine-α, is recognized by the carrot phytosulfokine receptor kinase, which is responsible for cellular dedifferentiation and proliferation in plants [6] . In prokaryotes, well-known sulfotransferases belong to the carbohydrate, aryl or glycolipid sulfotransferase families [7] , [8] , [9] , [10] . For example, the Sinorhizobium meliloti Nod factor (a lipo-chitooligosaccharide (LCO)), is sulfated by the NodH sulfotransferase, which transfers the sulfuryl group from 3′-phosphoadenosine 5′-phosphosulfate (PAPS) onto the Nod factor [7] , [11] . NodP and NodQ encode ATP sulfurylase and adenosine-5′-phosphosulfate (APS) kinase, which together catalyse the production of PAPS. S. meliloti strains carrying mutations in the nodP , nodQ or nodH genes, produce Nod factor that lacks the sulphate group and are severely impaired in their ability to nodulate their normal host alfalfa [7] . Tyrosine sulfotransferase activity has not previously been reported in prokaryotes [1] , [11] . We recently reported that the rice XA21 pattern recognition receptor binds a sulfated peptide (AENLSY S NFVEGDYVRTP; called axY S 22) derived from the Ax21 (activator of XA21-mediated innate immunity) protein present in the Gram-negative bacterium, Xanthomonas oryzae pv. oryzae ( Xoo ) strain PXO99 (refs 12 , 13 ). The biological function of Ax21 is to mediate quorum sensing (QS), a process where small molecules serve as signals to recognize cell population size, leading to changes in expression of specific genes when the QS factor has accumulated to a certain threshold concentration [14] , [15] . Ax21-mediated QS controls motility, biofilm formation and virulence in Xoo [13] , [14] . The Xoo genes raxST, raxP and raxQ, are also required for activation of XA21-mediated immunity. Xoo raxP and raxQ are predicted orthologs of S. meliloti nodP and nodQ, respectively. The raxST gene encodes a protein carrying a PAPS-binding motif [16] . Xoo mutant strains lacking ax21 (PXO99Δ ax21 ), raxST ( PXO99Δ raxST), raxP (PXO99Δ raxP ) or raxQ (PXO99Δ raxQ ) fail to activate XA21-mediated immunity [16] , [17] , [18] . The diverse Ax21-mediated biological activities in Xoo also require RaxST [14] . Based on the presence of the PAPS-binding motif in the raxST gene, we hypothesized that RaxST utilizes PAPS produced by RaxP and RaxQ to transfer a sulfuryl group (SO 3 −1 ) to Ax21. Using a newly developed sulfotransferase assay system, here we show that RaxST has tyrosine sulfotransferase activity. Furthermore, we provide direct evidence that Ax21 is a substrate of RaxST using ultraviolet photodissociation (UVPD) mass spectrometry. These studies demonstrate the occurrence of post-translational sulfation in a Gram-negative bacterium and further show the importance of sulfated proteins in triggering the host innate immune response and in bacterial cell–cell communication. PAPS is required for immune recognition of bacterial Ax21 To confirm the hypothesis that RaxST uses PAPS generated by RaxP and RaxQ to transfer a sulfuryl group (SO 3 −1 ) to Ax21, we tested if the raxQ knockout strain (PXO99 ΔraxQ ), which cannot make PAPS [17] , can be complemented by the addition of exogenous PAPS. XA21 rice leaves pretreated with the PXO99 ΔraxQ supernatant failed to induce XA21-mediated immunity and were susceptible to subsequent infection by PXO99 ΔraxST ( Supplementary Fig. S1 ). In contrast, rice leaves pretreated with PXO99 ΔraxQ supernatants from cultures that were incubated with exogenous PAPS are capable of inducing a robust immune response in XA21 plants. These pretreated XA21 plants are resistant to subsequent infection by PXO99 ΔraxST . This result indicates that RaxST utilizes PAPS produced by RaxQ. RaxST possesses sulfotransferase activity To test if RaxST carries tyrosine sulfotransferase activity, we generated biologically active, soluble recombinant RaxST ( Supplementary Fig. S2 ) and confirmed biological activity ( Supplementary Fig. S3 ). We then developed a system to measure sulfotransferase activity that relies on the measurement of NADPH production ( Fig. 1a ). This assay system was validated using a well-characterized human dopamine sulfotransferase, SULT1A3, and its substrate, dopamine ( Fig. 1b ). Next, we examined catalytic activity of RaxST using the N-terminal peptide of the CC-chemokine receptor 5, Y-peptide (DYQVSSPIYDINYYTSE), which is known to be a substrate for two human tyrosine sulfotransferases [19] . We found that NADPH production decreased when RaxST and the Y-peptide were added in the presence of limiting PAPS concentration ( Fig. 2a ). The reduction of NADPH was not observed in control reactions lacking either RaxST or the Y-peptide. These results indicate that RaxST has sulfotransferase activity. 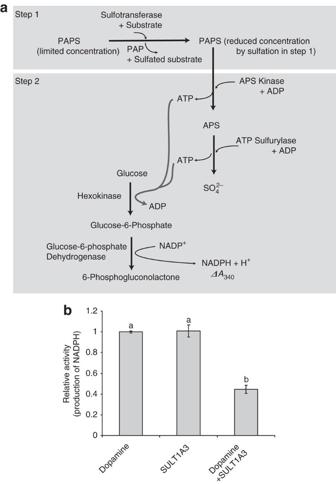Figure 1: Development of a sulfotransferase activity assay. (a) In the first step, a sulfotransferase, a substrate and PAPS are incubated under conditions that allow for the production of a sulfated substrate. In the next step, APS kinase and ATP sulfurylase catalyse reverse reactions to produce APS and ATP from the PAPS remaining from the first step. If PAPS is limiting, less APS and ATP will be produced. A subsequent reaction catalysed by hexokinase and glucose-6-phosphate dehydrogenase utilizes the ATP and glucose to produce the reduced form of nicotinamide adenine dinucleotide phosphate (NADPH) and 6-phosphogluconolactone. NADPH production can be specifically monitored at 340 nm using a spectrophotometer. In this assay system, two moles of NADPH are produced for each mole of PAPS turned over by APS kinase. Given an excess of PAPS and all other components in each step, the reaction rate will proceed in the absence of a sulfotransferase or its substrate (the sulfuryl-group receiver). If, however, an active sulfotransferase and substrate are incubated together before the addition of APS kinase under limited concentration of PAPS, NADPH production is decreased compared with that detected in reactions lacking a sulfotransferase or its substrate. This decrease reflects the presence of sulfotransferase enzymatic activity. Specific conditions are described in Methods. (b) Validation of the enzyme-coupling sulfotransferase assay system using dopamine sulfotransferase, SULT1A3 (25 units), and its substrate, dopamine (60 μM). NADPH production was measured at 340 nm using a spectrophotometer. Bars indicate the relative average value obtained for ΔA340/min±s.d. in three independent experiments. Different letters on the top of each bar indicate statistically significant differences between treatments ((one-way ANOVA analysis (Holm–Sidak test,P<0.05)). Figure 1: Development of a sulfotransferase activity assay. ( a ) In the first step, a sulfotransferase, a substrate and PAPS are incubated under conditions that allow for the production of a sulfated substrate. In the next step, APS kinase and ATP sulfurylase catalyse reverse reactions to produce APS and ATP from the PAPS remaining from the first step. If PAPS is limiting, less APS and ATP will be produced. A subsequent reaction catalysed by hexokinase and glucose-6-phosphate dehydrogenase utilizes the ATP and glucose to produce the reduced form of nicotinamide adenine dinucleotide phosphate (NADPH) and 6-phosphogluconolactone. NADPH production can be specifically monitored at 340 nm using a spectrophotometer. In this assay system, two moles of NADPH are produced for each mole of PAPS turned over by APS kinase. Given an excess of PAPS and all other components in each step, the reaction rate will proceed in the absence of a sulfotransferase or its substrate (the sulfuryl-group receiver). If, however, an active sulfotransferase and substrate are incubated together before the addition of APS kinase under limited concentration of PAPS, NADPH production is decreased compared with that detected in reactions lacking a sulfotransferase or its substrate. This decrease reflects the presence of sulfotransferase enzymatic activity. Specific conditions are described in Methods. ( b ) Validation of the enzyme-coupling sulfotransferase assay system using dopamine sulfotransferase, SULT1A3 (25 units), and its substrate, dopamine (60 μM). NADPH production was measured at 340 nm using a spectrophotometer. Bars indicate the relative average value obtained for Δ A 340 /min±s.d. in three independent experiments. Different letters on the top of each bar indicate statistically significant differences between treatments ((one-way ANOVA analysis (Holm–Sidak test, P <0.05)). 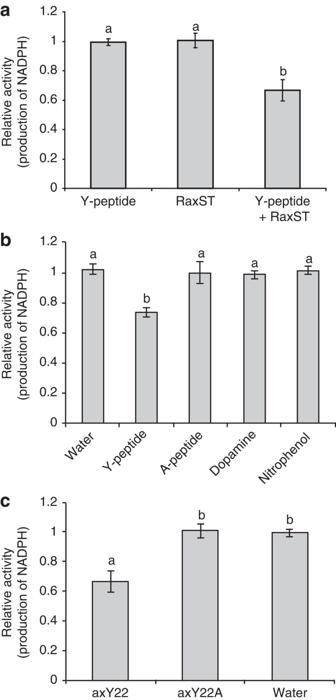Figure 2: (a) Tyrosine sulfotransferase activity of the RaxST protein. The reaction was initiated by adding the Y-peptide (DYQVSSPIYDINYYTSE) alone, RaxST protein alone, or both the Y-peptide and 0.5 μg of RaxST protein. (b) RaxST activity is specific to tyrosine peptides. The reaction was incubated with water, Y-peptide, A-peptide (DAQVSSPIADINAATSE), Dopamine or Nitrophenol. (c) RaxST activity is specific to axY22. The reaction was initiated by adding axY22, axY22A (AENLSANFVEGDYVRTP) or water. NADPH production was measured at 340 nm using a spectrophotometer. Bars indicate the relative average value obtained for ΔA340/min±s.d. in three independent experiments. Different letters on the top of each bar indicate statistically significant differences between treatments. (one-way ANOVA analysis (Holm–Sidak test,P<0.05)). Full size image Figure 2: (a) Tyrosine sulfotransferase activity of the RaxST protein. The reaction was initiated by adding the Y-peptide (DYQVSSPIYDINYYTSE) alone, RaxST protein alone, or both the Y-peptide and 0.5 μg of RaxST protein. ( b ) RaxST activity is specific to tyrosine peptides. The reaction was incubated with water, Y-peptide, A-peptide (DAQVSSPIADINAATSE), Dopamine or Nitrophenol. ( c ) RaxST activity is specific to axY22. The reaction was initiated by adding axY22, axY22A (AENLSANFVEGDYVRTP) or water. NADPH production was measured at 340 nm using a spectrophotometer. Bars indicate the relative average value obtained for Δ A 340 /min±s.d. in three independent experiments. Different letters on the top of each bar indicate statistically significant differences between treatments. (one-way ANOVA analysis (Holm–Sidak test, P <0.05)). Full size image SULT1A3 is known to utilize both dopamine and tyrosine as substrates [20] . To determine if the RaxST protein also has dual specificity, we tested nitrophenol and dopamine, which are known substrates of SULT1A2 and SULT1A3, respectively [20] , [21] . In addition, we also tested a variant of the Y-peptide in which the tyrosine residues were replaced with alanine residues (A-peptide, DAQVSSPIADINAATSE) to confirm whether the RaxST protein specifically targets tyrosine. The production of NADPH decreased only when the Y-peptide was added but not by the addition of the A-peptide, dopamine or nitrophenol ( Fig. 2b ), indicating that sulfation by RaxST is specific to a peptide-carrying tyrosine, not dopamine or nitrophenol as substrates. These results demonstrate that the RaxST protein specifically catalyses the sulfation of tyrosine residues. To determine optimal conditions for RaxST activity, we tested RaxST activity using the Y-peptide at different pH and temperatures. RaxST showed maximum activity at weak acidic conditions (approximately pH 6.5~6.8 and 25~30 °C)( Supplementary Fig. S4A and B ). A Michaelis–Menten plot was established to assess the kinetics of the reaction. Under the given conditions, the Km was 1.7 μM and the Vmax was 0.18 units mg −1 ( Supplementary Fig. S4C and D ). axY22 peptide sulfation is specifically catalysed by RaxST We next tested if RaxST can catalyse sulfation of axY22 and a peptide variant carrying alanine in place of the tyrosine in position 22 (axY22A, AENLSANFVEGDYVRTP). We found that production of NADPH decreased when axY22 was used as a substrate in the presence of RaxST and limiting concentrations of PAPS ( Fig. 2c ), indicating that axY22 is indeed a substrate for RaxST. By contrast, the peptide variant, axY22A, is not a substrate for RaxST, indicating that the Y-residue in position 22 is the only target of RaxST and not the additional tyrosine residue in position 29 ( Fig. 2c ). Taken together, these studies indicate RaxST catalyses sulfation of tyrosine 22 on the axY22 peptide to produce the biologically active form. Confirmation of sulfation of Ax21 by UVPD For a more direct determination of the RaxST target and to assess if other tyrosines are sulfated on the Ax21 protein, we expressed and purified the full-length mature Ax21 protein ( Supplementary Fig. S5 ) and subjected it to RaxST sulfation. We then purified the sulfated protein product, subjected it to GluC proteolytic digestion, and then analysed the resulting peptides via liquid chromatography-mass spectrometry (LC-MS/MS) in the negative nanoelectrospray mode with UVPD implemented on a Thermo Scientific Orbitrap Elite mass spectrometer. UVPD has proven to be a versatile MS/MS strategy for proteomics applications [22] , with particular merits for peptide anions for which conventional collision-induced dissociation (CID) and electron-based activation methods (ECD, ETD) are less successful [23] , [24] . Tyrosine sulfation is a particularly labile modification upon CID of protonated or deprotonated peptides [25] , making UVPD a compelling alternative. Here we demonstrate the first application of the UVPD approach for assessment of tyrosine sulfation. Despite the low abundance of the peptide in the Ax21 digest, the UVPD fragmentation pattern ( Fig. 3 ) confidently confirmed the sequence (NSLYNFVE) and sulfation site (Y22) with diagnostic a 5 , a 6 , a 7 , x 7 and x 8 ions and retention of the modification on all of the key sequence ions. The ion assignments and mass accuracies corresponding to Fig. 3 are summarized in Supplementary Table S1 , and the negative UVPD mass spectrum of a synthetic sulfated model peptide is displayed in Supplementary Fig. S6 . The sulfation modification was not successfully identified using the more conventional CID and ETD methods in the positive ionization mode for tryptic or GluC digests of the Ax21 protein. 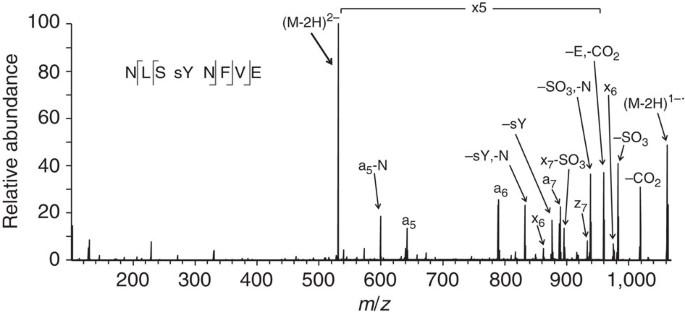Figure 3: UV photodissociation mass spectrum of Tyr-sulfated peptide NLSYNFVE. The Tyr-sulfated peptide was identified in the GluC digest of Ax21 after incubation with the sulfotransferase RaxST. The spectrum of the doubly deprotonated (2−) peptide was acquired on an Orbitrap Elite mass spectrometer equipped with an excimer laser (193 nm, 500 Hz, 5 ns pulse, 2 mJ per pulse, two pulses per spectrum). UVPD occurred in the higher-energy collisional dissociation (HCD) cell of the Orbitrap Elite mass spectrometer. Figure 3: UV photodissociation mass spectrum of Tyr-sulfated peptide NLSYNFVE. The Tyr-sulfated peptide was identified in the GluC digest of Ax21 after incubation with the sulfotransferase RaxST. The spectrum of the doubly deprotonated (2−) peptide was acquired on an Orbitrap Elite mass spectrometer equipped with an excimer laser (193 nm, 500 Hz, 5 ns pulse, 2 mJ per pulse, two pulses per spectrum). UVPD occurred in the higher-energy collisional dissociation (HCD) cell of the Orbitrap Elite mass spectrometer. Full size image Post-translational modifications of prokaryotic proteins are poorly understood compared with those of eukaryotes. The discovery of tyrosine sulfation of Ax21 by RaxST represents a previously unreported post-translational modification in bacteria and provides new insight into the role of such a modification in triggering the host innate immune response and in controlling bacterial cell–cell communication. Biological materials Bacterial strains and plasmids used in this study are listed in Supplementary Table S2 . Sulfotransferase activity assay Unless otherwise indicated, reactions were initiated by adding a sulfotransferase and its substrate at the desired concentration in 50 μl of sulfotransferase buffer (8 μM PAPS, 10 mM Tris–HCl, pH 7.0, 1 mM adenosine monophosphate, 50 mM NaF, 0.5% Triton-100 and 5 mM MnCl 2 ). Sulfotransferase buffer was freshly prepared for each experiment. After 4 h of incubation at 30 °C, the reaction mixture was chilled on ice. The APS cocktail buffer contained 50 mM Tris–HCl, pH 7.0, 70 mM (NH 4 ) 2 SO 4 , 5 mM MgCl 2 , 0.6 mM nicotinamide adenine dinucleotide phosphate (NADP + ), 1 mM glucose, 1 mM sodium pyrophosphate, 560 μM adenosine diphosphate, 2.5 units of glucose-6-phosphate dehydrogenase, 5 units of hexokinase, 55 μg of ATP sulfurylase and 8 μg of APS kinase. The construct containing APS kinase in the pET15b vector was kindly provided by Dr Andrew Fisher at UC Davis. We purified APS kinase from E. coli expressing the His-tagged APS kinase fusion protein using an Ni-NTA agarose column and tested its activity using a previously established method [26] . All other co-enzymes and chemicals were purchased from Sigma. For each assay, 50 μl of APS cocktail buffer was added to the ice-chilled sulfotransferase reaction mixture. The coupling assay was finally initiated by adding APS kinase. NADPH production was measured using a SafireII spectrophotometer (Tecan) at 340 nm and 30 °C at 30-s intervals. In the figures, the relative activity of the y axis refers to the amount of NADPH produced at a specific time point (7 min after the addition of APS kinase). The values are relative to the controls (water or sulfotransferase only), which were set as one. Enzymatic analysis of RaxST To assay the enzymatic activity of RaxST, 0.15 or 0.45 μg of the partially purified RaxST and 100 μM synthetic tyrosine peptide (NH 2 -DYQVSSPIYDINYYTSE, referred to as Y-peptide) were used. To assess the specificity of tyrosine sulfotransferase activity, we generated another peptide in which all the tyrosine residues in the Y-peptide were replaced with alanine (NH 2 -DAQVSSPIADINAATSE, referred to as A-peptide). In addition, dopamine (1.92 mM) and nitrophenol (640 μM) were tested using the sulfotransferase enzyme-coupling assay described above. To determine the optimum conditions for RaxST activity, RaxST and Y-peptide were incubated at 6, 16, 30 or 37 °C and at pH 5, 6, 7 or 8 in 10 mM MES, HEPES or Tris–HCl buffer at 30 °C. Following the reaction with RaxST and Y-peptide, the resultant APS kinase activity was monitored at 30 °C, pH 7.0. For kinetic analysis of RaxST with Y-peptide, we used 0, 0.5, 1, 2.5, 5, 10, 25, or 50 μM Y-peptide. The K m and V max values were determined using a double reciprocal plot. Ax21 is a substrate of RaxST To test if peptide axY22 is a substrate of RaxST, we generated two peptides based on the amino-acid sequence of the Ax21 protein (AENLSYNFVEGDYVRTP, axY22, and AENLSANFVEGDYVRTP, axY22A). The reaction was initiated by adding 0.45 μg of partially purified RaxST protein and 100 μM axY22 or axY22A in 50 μl of sulfotransferase buffer. After 4 h of incubation at 30 °C, the reaction mixture was chilled on ice. A total of 50 μl of APS cocktail buffer was added to the ice-chilled sulfotransferase reaction mixture. The coupling assay was finally initiated by adding APS kinase. NADPH production was measured using a SafireII spectrophotometer (Tecan) at 340 nm and 30 °C. To determine if the mature Ax21 protein also serves as substrate for RaxST and if other tyrosine residues could serve as sites for RaxST-mediated sulfation, we used E. coli -purified Ax21 and RaxST. We incubated 20 μg of RaxST with 200 μg highly purified MBP-Ax21 fusion in freshly made sulfation buffer (25 mM Tris pH 7.5, 150 mM NaCl, 20 mM MgCl 2 , 480 μM PAPS) for 4 h at 30 °C. Samples were then kept on dry ice, or −80 °C until analysed by LC-MS/MS. Sample preparation for LC-MS/MS analysis A total of 20 μg of the RaxST/MBP-Ax21 fusion protein mixture was prepared for digestion by performing a buffer exchange using a 10-KDa molecular weight cut-off filter. The filtered protein was diluted in 1% Protease Max (Promega) in 1 × phosphate-buffered saline. The protein was reduced with dithiothreitol for 30 min (55 °C), then incubated with iodoacetamide at room temperature for 30 min in the dark. For GluC digestion, 1 μl of 1 μg μl −1 GluC protease in water was added, giving a protein to enzyme ratio of 20:1. The digestion solution was incubated for 4 h at 37 °C. For trypsin digestion, 1 μl of trypsin (1 μg μl −1 ) was added to 20 μg of buffer exchanged, reduced and alkylated protein solution and incubated overnight at 37 °C. Following digestion, the solutions was desalted using C18 spin columns (Thermo/Pierce) and reconstituted in 98% water, 2% acetonitrile for LC-MS/MS analysis. LC-MS/MS and UVPD analysis LC-MS analysis was undertaken using a Dionex Ultimate 3000 RSLC system operated in a reversed phase nano-liquid chromatography mode at a flow rate of 300 nl min −1 . A total of 3 μl of the GluC digest was injected onto a New Objective IntegraFrit 100-μm inner diameter trap column (Woburn, MA) packed with Michrom Magic C18 AQ (Auburn, CA) to 3.6 cm. Samples were preconcentrated for 3 min using 2% acetonitrile/0.05% acetic acid at a flow rate of 5 μl min −1 . The preconcentration column was then switched in-line with a New Objective PicoFrit analytical column (Woburn, MA) (75 μm × 20 cm) packed with 5 μm Michrom Magic C18 AQ. Separation was performed with eluent A consisting of 0.05% acetic acid in water and eluent B consisting of 0.05% acetic acid in acetonitrile with a 140-min linear gradient from 3 to 30% eluent B at a flow rate of 300 nl min −1 . Mass spectrometric analysis was performed on a Thermo Scientific Orbitrap Elite mass spectrometer (Thermo Fisher Scientific, Bremen, Germany) equipped with a Coherent (Santa Clara, CA) ExciStar XS excimer laser (Coherent Inc., Santa Clara, CA) operated at 193 nm. The coupling of the laser to an orbitrap mass spectrometer was described in detail previously [27] . Data-dependent nanoLC-MS/UVPD was performed as follows: the first event was the survey-negative mass scan ( m/z range of 400–2,000) at resolution 120,000 (1 μscan) followed by ten UVPD events on the ten most abundant ions from the survey scan at resolution 15,000. The isolation width was set to 2.00 and the minimum required signal was 4,000.00. Dynamic exclusion settings included a repeat count of 1 during a 30.00 s timeframe. The exclusion duration was 60.00 s. Exclusion mass width relative to low and high (p.p.m.) was set to 10. A series of two 2 mJ UV pulses (applied during a 4-ms activation period) was used per MS/MS scan with normalized collision energy set to 1. One μscan was performed per MS/MS scan. After an initial run in which the entire range was monitored in a data-dependent manner and the elution of the sulfated peptide ( m / z 531) was identified, the mass spectrometer was then set to monitor m / z 531 and to perform UVPD for increased sensitivity during the elution range of 40 and 105 min. All spectra were processed using the MassMatrix database search engine. The LC-MS CID method incorporated the same survey scan and dynamic exclusion parameters described above followed by a series of top ten data-dependent scans for which an isolation width of 2 was used and the minimum required signal was 8,000.0. Normalized collision energy for CID was 35.0 with an activation q of 0.250. The number of microscans was set to 1. In the negative mode, the FTMS full AGC target was 1,000,000.00 and the FTMS MSn AGC target was 50,000.00. The maximum ion time was 500.00 ms for FTMS full and MSn scans. The source voltage was 1.60 kV and the capillary temperature was 275 °C. In the positive mode, the FTMS full AGC target was 1,000,000.00 and the ion-trap MSn AGC target was 10,000.00. The maximum ion time was 100 ms and 200 ms for FTMS full- and ion-trap MSn scans. The source voltage was 1.70 kV and the capillary temperature was 275 °C. Accession codes: The mass spectrometry data have been deposited in Peptide Atlas under accession codes PASS00077, PASS00078, and PASS00079. How to cite this article: Han, S-W. et al. Tyrosine sulfation in a Gram-negative bacterium. Nat. Commun. 3:1153 doi: 10.1038/ncomms2157 (2012).